Electrochemical dynamics of nanoscale metallic inclusions in dielectrics Nanoscale metal inclusions in or on solid-state dielectrics are an integral part of modern electrocatalysis, optoelectronics, capacitors, metamaterials and memory devices. The properties of these composite systems strongly depend on the size, dispersion of the inclusions and their chemical stability, and are usually considered constant. Here we demonstrate that nanoscale inclusions (for example, clusters) in dielectrics dynamically change their shape, size and position upon applied electric field. Through systematic in situ transmission electron microscopy studies, we show that fundamental electrochemical processes can lead to universally observed nucleation and growth of metal clusters, even for inert metals like platinum. The clusters exhibit diverse dynamic behaviours governed by kinetic factors including ion mobility and redox rates, leading to different filament growth modes and structures in memristive devices. These findings reveal the microscopic origin behind resistive switching, and also provide general guidance for the design of novel devices involving electronics and ionics. The ability to control and manipulate metal inclusions (for example, individual metal clusters) inside a solid-state medium will greatly expand the functions and create new classes of materials (for example, metamaterials) and devices for electronic, magnetic, photonic, chemical and optoelectronic applications [1] , [2] , [3] , [4] , [5] , [6] . Such abilities have been demonstrated, for example, with scanning tunneling microscopy tools [1] . However, manual manipulation using scanning tunneling microscopy is slow and inefficient, and not device-friendly compared with methods such as using local electric fields. Indeed, devices based on the field-driven migration of metal inclusions (such as resistive switching or memristive devices) [7] , [8] , [9] have attracted broad interest recently and have shown great potential as a disruptive technology for a number of applications including nonvolatile memory [10] , [11] , [12] , [13] , logic [14] , [15] , [16] and neuromorphic computing [17] . In these devices, the resistive switching is normally attributed to filament formation caused by the movement of metal inclusions in the insulating dielectric film [9] , [10] , [18] , [19] , [20] . Attempts to microscopically study the filament growth processes have been carried out using scanning probe microscopy [15] , [21] and high-resolution transmission electron microscopy [19] , [20] , [22] , [23] , [24] techniques. For example, a recent experiment reveals different filament growth modes [20] and shows that filament formation can be achieved in the form of metal nanoclusters. However, a critical question was raised regarding the fundamental, microscopic origin of the growth and migration of the nanoclusters inside dielectrics [25] , and whether the different and seemingly contradicting experimental results can be reconciled within the same theoretical framework. Here we directly reveal the microscopic origin of the dynamic growth and migration processes of metal nanoclusters in dielectrics and show that the field-driven migration is a universal behaviour, even for inert metals such as Pt. We show the different migration modes can be explained in the electrochemical model framework, driven by both thermodynamic and kinetic factors. Specifically, we show that in conventional insulators the metal clusters can be treated as bipolar electrodes (BPEs), and can dissolve from their original locations and nucleate and redeposit at new positions closer to the counter electrode in a process driven by the competing electrochemical processes occurring at the two polarized sides. We show this fundamental process can be used to explain the diverse filament growth modes observed experimentally, and predict and verify the growth modes at different limiting cases, therefore reconciling the different experimental results obtained earlier within a generalized theoretical framework [10] , [20] , [22] . By tuning kinetic factors, we further show different nanocluster dynamics can be observed in the same device, leading to the transition between different filament growth modes. Dynamic migration of metal nanoclusters In situ transmission electron microscopy (TEM) studies were first conducted on bulk samples consisting of individual metal nanoclusters embedded in the bulk of a dielectric film. This approach enables detailed analysis and tracking of individual clusters and ensures the migration occurs inside the bulk of the film. By tracing the dynamic motion of the same nanocluster under electric field in an in situ TEM setup for different material systems (Ag, Cu, Pt, Ni), we successfully revealed fundamental atomic/ionic dynamics that are universally applicable. The experimental strategy is illustrated in Fig. 1a–d , using Ag nanoclusters as an example. An array of Ag nanoclusters was embedded inside the SiO 2 film by annealing a stacked SiO 2 /Ag/SiO 2 structure with a ~\n1-nm-thin Ag layer. Inert Au electrodes were then deposited to apply electric fields across the SiO 2 /Ag/SiO 2 stack (see Methods). SiO 2 was selected as the dielectric layer in this study because it is the most important dielectric material in the semiconductor industry and is also widely used for other devices including memristive devices [18] , [26] , [27] . Successive focused ion beam (FIB) lift-out, patterning, and thinning processes were subsequently performed to prepare an array of Au/SiO 2 /Ag nanoclusters/SiO 2 /Au devices with individual top electrodes and shared bottom electrode for cross-sectional TEM studies ( Fig. 1b–d ). During in situ TEM analysis, the top Au electrode of a device is contacted by a movable W probe, whereas the bottom Au electrode is grounded ( Fig. 1d ). 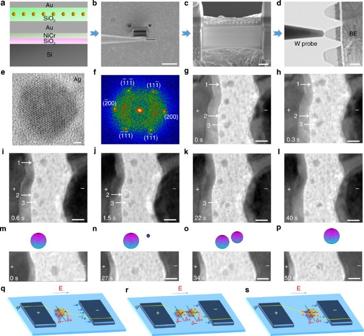Figure 1: Dynamic growth and migration of Ag nanoclusters in a dielectric film. (a) Schematic of the samples consisting of Ag nanoclusters embedded in a SiO2film. The field was applied through the Au electrodes. (b) Scanning electron microscopy (SEM) image showing the FIB lift-out process. Scale bar, 20 μm. (c) SEM image showing an array of samples prepared by FIB. Scale bar, 1 μm. (d) TEM image showing thein situexperimental setup. Scale bar, 200 nm. (e) High-resolution transmission electron microscopy image and (f) corresponding fast Fourier transformation (FFT) results showing the single-crystalline face-centered cubic (fcc) structure of a Ag nanocluster. Scale bar, 1 nm. (g–l) Real-time TEM images capturing the growth and migration of Ag nanoclusters under electric field. Scale bar, 10 nm. (m–p)In situTEM images along with simulation results showing the dissolution and growth processes between two Ag nanoclusters. Scale bar, 10 nm. (q) Schematic of a polarized Ag nanocluster embedded in SiO2under electric field, overlaid with the electric potential. (r) New cluster nucleation and formation of another bipolar electrode nearby. (s) The dissolution of the original cluster and the growth of the new cluster lead to an effective movement of a cluster along the electric field. Figure 1e shows a TEM image of one of the embedded Ag nanoclusters along its [011] zone axis, with the corresponding fast Fourier transformation results displayed in Fig. 1f , which clearly reveal the crystalline face-centered cubic structure of the Ag cluster. Figure 1: Dynamic growth and migration of Ag nanoclusters in a dielectric film. ( a ) Schematic of the samples consisting of Ag nanoclusters embedded in a SiO 2 film. The field was applied through the Au electrodes. ( b ) Scanning electron microscopy (SEM) image showing the FIB lift-out process. Scale bar, 20 μm. ( c ) SEM image showing an array of samples prepared by FIB. Scale bar, 1 μm. ( d ) TEM image showing the in situ experimental setup. Scale bar, 200 nm. ( e ) High-resolution transmission electron microscopy image and ( f ) corresponding fast Fourier transformation (FFT) results showing the single-crystalline face-centered cubic (fcc) structure of a Ag nanocluster. Scale bar, 1 nm. ( g – l ) Real-time TEM images capturing the growth and migration of Ag nanoclusters under electric field. Scale bar, 10 nm. ( m – p ) In situ TEM images along with simulation results showing the dissolution and growth processes between two Ag nanoclusters. Scale bar, 10 nm. ( q ) Schematic of a polarized Ag nanocluster embedded in SiO 2 under electric field, overlaid with the electric potential. ( r ) New cluster nucleation and formation of another bipolar electrode nearby. ( s ) The dissolution of the original cluster and the growth of the new cluster lead to an effective movement of a cluster along the electric field. Full size image When an electric field is applied, evolution and migration of the embedded Ag nanoclusters can be regularly observed, as shown in Fig. 1g–l (also see Supplementary Movie 1 ). The nanoclusters have diameters of ~\n5 nm and the applied voltage was 3 V corresponding to an electric field of ~\n0.8 MV cm −1 . Notably, at location 1 (marked by the upper arrow) dynamic interactions between a pair of Ag nanoclusters were observed. As shown in Fig. 1g–i , the cluster on the left (upstream in the direction of the electric field) was gradually dissolved and merged into another cluster on the right side (downstream), resulting in an overall movement of Ag clusters along the direction of the applied electric field. Similarly, clusters 2 (marked by the middle arrow) and 3 (marked by the lower arrow) were also gradually dissolved. Cluster 2 disappeared ( Fig. 1k ) and left a void in the film as shown in Fig. 1j,k . Additionally, as cluster 3 was dissolved a new cluster, named cluster 4, emerged nearby, as marked by the lower circle in Fig. 1k,l . These behaviours have been repeatedly observed in different devices. Figure 1m–p shows the interactions between another pair of Ag nanoclusters, and illustrates the gradual dissolution of the original cluster upstream and the nucleation and growth of another cluster downstream. The original Ag cluster was completely dissolved and left a void behind in the original position (marked by circle in Fig. 1p , see Supplementary Movie 2 ), and effective growth along the field direction was achieved. The dynamic evolution of metal nanoclusters revealed by in situ TEM can be consistently explained in the theoretical framework of electrochemical redox processes in BPEs with strong influence from kinetic effects. Under an electric field inside the dielectric, the metal nanoclusters can be treated as BPEs [25] , [28] , [29] , with an effective cathode (δ–) facing the field direction and an effective anode (δ+) on the opposite side, as shown in Fig. 1q . In this model, Ag + ions will be generated from the anode side of the clusters via electrochemical oxidation processes. The Ag + ions will drift along the electric field and become reduced when they reach a cathode (for example, the cathode side of another Ag cluster downstream). In the current experimental setup, there is no Ag supply to the first Ag cluster upstream, so it experiences only net oxidation and thus gradually dissolves. The created Ag + ions can be reduced and deposit onto the second nanocluster downstream. If oxidation on the anode side of the 2nd nanocluster is suppressed (due to, for example, kinetic limitations discussed later), the 2nd nanocluster will experience net growth. As a result, the first cluster merges into the 2nd nanocluster downstream, resulting in an effective cluster displacement along the electric field, as shown in Fig. 1q–s . It is worthwhile noting that charge neutrality needs to be maintained in the nanocluster after the generation of Ag + ions. The possible processes involve reduction of another Ag + ion at the cathode side of the BPE, escape of the trapped electron, or through another reaction process (for example, reduction of moisture or proton [27] ). In addition, the redox and migration processes of a specific cluster are determined by the local electrochemical and/or structural environment sensed by the cluster and are affected by the film inhomogeneity and electric field distribution, so the cluster dynamics are stochastic in nature. For example, out of the five Ag clusters shown in Fig. 1g–i , the three marked clusters migrated to different new locations at different times, while the other two clusters did not undergo apparent oxidation processes within the measurement time frame. We note the formation of the 2nd nanocluster inside the SiO 2 film requires first a nucleation process, that is, the initial formation of a critical nucleus. This process can be regarded as a chemical process of formation of stable atomic configuration to minimize the excess surface energy and allow further growth. The free enthalpy of nucleation is given by [30] : Where N c is the number of atoms constituting the critical nucleus; Δ G is the free enthalpy of nucleation; Δ φ is the voltage drop (a part of the applied voltage, depending on the position of the nucleus); Φ the surface energy contribution and ε is the strain energy per atom. Δ φ , Φ and ε will have significant influence on the nucleation as a function of the particular local chemical, electrical and mechanical properties of the oxide matrix. As a result, the nucleation process is spatially selective instead of being homogenous, as shown in Fig. 1 and Supplementary Movies 1–4 . If nucleation could not proceed, the Ag + ions can reach the Au counter electrode and become reduced there. This appears to be the case for cluster 2 in Fig. 1g–l . However, a significant geometric change may not be observed in this case due to the much larger volume of the electrode. These analyses show that kinetic factors (for example, the interplay between the redox rates at the cathode/anode sides of the BPE, nucleation rates and ionic migration speed) of the electrochemical redox reactions and ionic drift strongly influence the dynamics of the metal nanoclusters. The evolution of the shape and size of a cluster can be determined by the competition between the oxidation and reduction rates on the cathode and anode sides of the BPE, which can be described as where V i is the volume of cluster i , and ( ) is the oxidation (reduction) rate for the Ag atoms (ions) on the anode and cathode sides of cluster i , respectively. For two neighbouring clusters ( i and i −1) with small distance, we can approximate the ion exchange as accounting for the conservation of the Ag material. In systems with more clusters interacting electrostatically, the different growth rates will be affected by the distance between the clusters, their relative position to each other and their sizes. These factors account for the electric field strength and the overall evolution of the system (for example, the conducting filament in a memristive device [20] ). In light of the above understandings, the experimental results that the clusters upstream merge into their counterparts downstream, for example, clusters 1 and 3 in Fig. 1g–l and the cluster in Fig. 1m , can be explained. Figure 1m–p shows simulation results using equations (2, 3) by assuming for the 2nd nanocluster (Methods). The simulation confirms the experimental observations ( Fig. 1m–p ). Other behaviours can also be expected from equation (2), as will be elaborated later. As the electric field is continuously applied, the cluster splitting and merging processes can be repeated, resulting in an effective displacement (movement) of the clusters along the electric field ( Fig. 1s ) towards the counter electrode. Since SiO 2 is an amorphous insulator rather than a homogeneous electrolyte, the conditions for ion migration and nucleation are inhomogeneous and depend strongly on the local microstructure, electric field distribution, electrochemical environment and presence of defects, as observed in Fig. 1g–p . We have extensively studied the behaviours of different metal systems, including active metals such as Ag and Cu as well as inert metals such as Ni and Pt. The volume of the source material was also varied systematically. Among these materials, Ag and Cu are widely recognized as the material of choice for the formation of metal filaments and most commonly used in resistive memory devices [9] , [10] , [12] , [18] . Compared with Ag, in situ TEM studies on Cu have shown essentially similar results. As displayed in Fig. 2a–f , after applying a voltage of 6 V, 3 Cu clusters were found to have nucleated and grown between the embedded Cu source and the counter Au electrode ( Fig. 2b , Supplementary Movie 3 ). As the sizes of the newly formed clusters 1–3 grew larger, these clusters also became oxidized ( Fig. 2c–f ), since the polarization strength of the clusters ( P ) are proportional to the cluster radius ( r ), that is, P = E · r (cos θ −cos λ ) (where θ and λ are angles used to define the position on the cluster surface) [25] . The electrochemical processes of the clusters thus enter a second stage and > applies. While clusters 1 and 2 were gradually dissolved, cluster 3 underwent another splitting→merging process and grew into cluster 4 that was even closer to the counter electrode. The dynamic behaviours of clusters 3 and 4 highlight the rapidly evolving kinetics of the BPEs, including < during initial growth ( Fig. 2b ), and subsequent transitions to > during the dissolution process ( Fig. 2c–f ). Significantly, these processes lead to a step-by-step movement of the metal inclusions along the electric field direction, and reveal the microscopic nature of the formation and dissolution processes of conducting filaments in dielectrics. 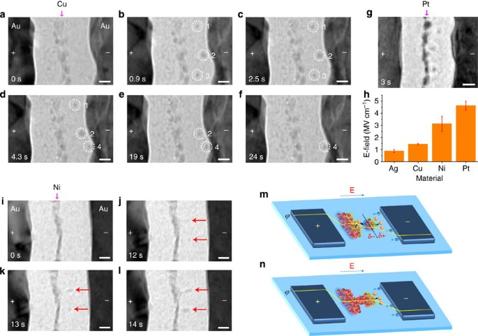Figure 2: Universal dynamic behaviours observed with different metal nanoclusters. (a–f)In situTEM images showing the movement of Cu nanoclusters under electric field. Scale bar, 10 nm. (g) TEM image showing the nucleation of Pt nanoclusters. Scale bar, 10 nm. (h) Distribution of the electric field required to drive the dissolution/nucleation processes for different materials. (i–l)In situTEM images showing the evolution of Ni nanoclusters. Scale bar, 10 nm. (m) Schematic of cluster nucleation from a large embedded metal source. (n) Schematic of the backward growth from the nucleus due to high ion concentration, forming a solid connection with the source. Figure 2: Universal dynamic behaviours observed with different metal nanoclusters. ( a – f ) In situ TEM images showing the movement of Cu nanoclusters under electric field. Scale bar, 10 nm. ( g ) TEM image showing the nucleation of Pt nanoclusters. Scale bar, 10 nm. ( h ) Distribution of the electric field required to drive the dissolution/nucleation processes for different materials. ( i – l ) In situ TEM images showing the evolution of Ni nanoclusters. Scale bar, 10 nm. ( m ) Schematic of cluster nucleation from a large embedded metal source. ( n ) Schematic of the backward growth from the nucleus due to high ion concentration, forming a solid connection with the source. Full size image In general, and can be impacted by many factors such as material properties, local electric field, the amount of available atoms/ions and charge compensation. As a result, complex electrochemical dynamics are expected, which could in turn lead to significantly different filament growth behaviours that explain the contradicting reports in the literature [10] , [20] , [22] , [25] . For example, in our experiments, the Pt clusters that were formed after the first nucleation process ( Fig. 2g ) were never found to be dissolved again within the time frame of the in situ experiments, probably due to the low for the newly formed Pt clusters. In another case for Ni clusters, persistent reduction of Ni ions (supplied from the large Ni source) onto the cathode side of an existing Ni cluster led to a backward growth towards the Ni source, as shown in Fig. 2i–l (also see Supplementary Movie 4 ). Since the volume of the Ni source was hardly changed, the deposition of the Ni ions leads to a backward connection between the nanocluster BPE and the Ni source ( Fig. 2n ). It should be noted that the backward growth in this case is still different from the conventional electrochemical metallization (ECM) model [10] , [12] , [18] , as the reduction process does not initiate from the counter electrode but instead from a BPE inside the dielectric. As a result, the filament will form an extension of the anode instead of the cathode as predicted by the ECM model. We have investigated dozens of devices based on different materials, and found it to be universally true that the apparent movements of metal nanoclusters are always along the direction of the electric field ( Figs 1 and 2 ). Different electric fields, however, are required for the migration of different metals within the measurement time frame of several minutes, as shown in Fig. 2h for Ag, Cu, Ni and Pt. The dissolution/nucleation of embedded Ag clusters inside SiO 2 was found to be the easiest, typically requiring an electric field of <1 MV cm −1 , while the electric field required for Cu movement is slightly higher but roughly in the same level. In contrast, the more inert Ni and Pt clusters require much higher electric field of 3–5 MV cm −1 . The different electric fields required for the cluster migration reflect the electrochemical activity of the different metals and this observation explains why Ag and Cu are more suitable for metal filament-based memristive devices [9] , [10] , [12] , [18] . In general, the ease of displacement of nanoclusters shows a tendency to increase as a function of the polarizability of the half-cell reaction, that is, the Ag + /Ag redox reaction is typically considered in liquid electrolytes as ideally non-polarizable, whereas the polarizability increases in the series Cu→Ni→Pt. Moreover, Ni- and Pt-ions have higher charge numbers and sizes, and their diffusion in solids is suppressed in contrary to Ag- and Cu-ions being well known as one of the most mobile ions in solids. Filament growth dynamics The controlled migration of nanoclusters can be used to design and tune the operations of novel electric devices. For example, memristive devices are based on the formation of conductive filaments and the insight gained from the migration of discrete metal nanoclusters naturally explains the filament growth dynamics in memristive devices. Specifically, the different filament growth modes observed experimentally [20] , [22] can now be reconciled in the same theoretical framework. In a simplified, qualitative model, the filament growth dynamics may fall into four different regimes depending on the kinetic factors. When the ion mobility ( μ ) and the redox rates Γ i are high and homogeneous (case a), the ions can reach the inert electrode without agglomerating, thus avoiding nucleation within the insulating film so filament growth initiates from the inert electrode, and the large amount of ion supply (due to high Γ i ) leads to an inverted cone-shaped filament [12] , [18] with its base at the inert electrode interface, as schematically shown in Fig. 3a . This is in agreement with the filament growth in conventional ECM devices, and corresponds to material systems with high ionic conductivity (that is, large amounts of ions and high ion mobility). An experimental proof for case a is the in situ TEM observation on devices based on Cu–GeTe electrolyte [22] . In contrast, in the other extreme of low and inhomogeneous μ and low Γ i (case b, Fig. 3b ), the ions can pile and reach the critical nucleation conditions inside the dielectric and further filament growth is fulfilled by cluster displacement via the repeated splitting→merging processes shown in Fig. 1 . An experimental example is the filament growth in amorphous Si, where the filament is initiated from the active electrode and grows towards the inert electrode as discrete nanoclusters [20] . This case corresponds to material systems with very low ionic conductivity. Instead, if the ion mobility is low while the redox rates are high (case c), nucleation can occur inside the dielectric while large amounts of atoms can be deposited onto the cathode sides of the nuclei, leading to gap filling shown in Fig. 3c . This case corresponds to observations in Fig. 2i–l . After a connection between the nuclei and the active electrode is made, the process is repeated thus again leading to an effective forward growth towards the inert electrode. Finally, if the ion mobility μ is high while the redox rates Γ i are low (case d), nucleation only occurs at the counter electrode but the limited ion supply means reduction predominately occurs at the edges with high field strengths, thus leading to branched filament growth towards the active electrode, as shown in Fig. 3d . This case corresponds to the experimental observations in sputtered SiO 2 films [20] , whose open structure and high defect density result in higher μ than evaporated SiO 2 . The different experimental observations can thus be fully accounted for in this generalized framework based on fundamental electrochemical processes. In general, the ion mobility in a given dielectric μ determines the nucleation sites and the direction of the filament growth, while the redox rates Γ i determine the ion supply and the geometry of the filament. By tuning these kinetic factors, different growth modes and filament geometry can be potentially controlled in a systematic fashion. In practice, the local μ and Γ i can be affected by variations in the local defect density, defect energy profile and local electrochemical potentials so different migration modes may be observed simultaneously in the same system. 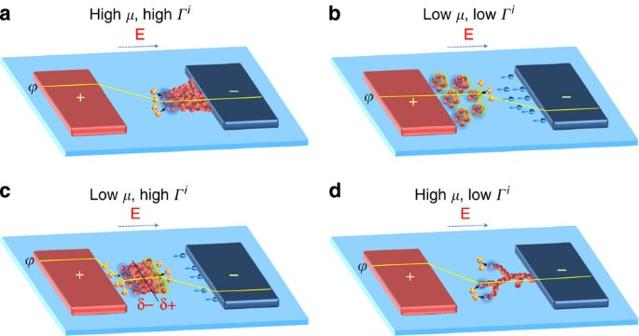Figure 3: Qualitative model showing filament growth dynamics governed by kinetic parameters. (a) Bothμand Γiare high, resulting in filament growth from the inert electrode and an inverted cone shape. (b) Bothμand Γiare low, resulting in filament growth from the active electrode with discrete nanoclusters and a forward cone shape. (c)μis low but Γiis high, resulting in filament nucleation inside the dielectric and reconnection with the source. (d)μis high but Γiis low, resulting in filament growth from the inert electrode and a branched structure. Figure 3: Qualitative model showing filament growth dynamics governed by kinetic parameters. ( a ) Both μ and Γ i are high, resulting in filament growth from the inert electrode and an inverted cone shape. ( b ) Both μ and Γ i are low, resulting in filament growth from the active electrode with discrete nanoclusters and a forward cone shape. ( c ) μ is low but Γ i is high, resulting in filament nucleation inside the dielectric and reconnection with the source. ( d ) μ is high but Γ i is low, resulting in filament growth from the inert electrode and a branched structure. Full size image To experimentally verify the theory, we performed in situ TEM studies in actual resistive memory structures. The devices consist of a Ag/SiO 2 /W structure with an evaporated SiO 2 film covering a W probe. Compared with sputtered SiO 2 , the evaporated SiO 2 here has less defects and lower μ , therefore this system in general falls into the low μ , low Γ i regime. The device was directly formed inside the TEM column by connecting a high-purity Ag wire with a movable W probe coated with the SiO 2 film ( Fig. 4a , Methods). Representative results for a device with a ~\n40-nm-thick SiO 2 film are shown in Fig. 4b–e (also see Supplementary Movie 5 ). The first visible filament growth in the SiO 2 film was the appearance of several Ag clusters near the Ag electrode after ~\n3 min ( Fig. 4b ). This is in agreement with the nucleation of metal nanoclusters in Figs 1 and 2 . These clusters then behave as BPEs during subsequent growth. As expected, over time these clusters move closer to the inert electrode, following the splitting→merging processes discussed earlier ( Fig. 1m–p ) and correspond to case b. Due to the higher concentration of Ag + ions near the Ag electrode and therefore the higher probability to overcome the nucleation barrier, more Ag clusters will be nucleated near the Ag electrode inside SiO 2 and the repeated nucleation and growth leads to the filament shape as observed Fig. 4d . As predicted for case b, this growth mode leads to a conically shaped filament ( Fig. 4d,e ) with its base at the Ag/SiO 2 interface and expanding towards the inert electrode. Such growth direction is in contrast to the conventional ECM growth model for solid electrolytes [10] , [18] but can be explained by the generalized framework discussed above. The overall growth of the filament can be then characterized by the step-by-step movements of Ag cluster components driven by the electrochemical kinetics, as illustrated by Fig. 4f–j (more details can be found in Supplementary Note 1 ). 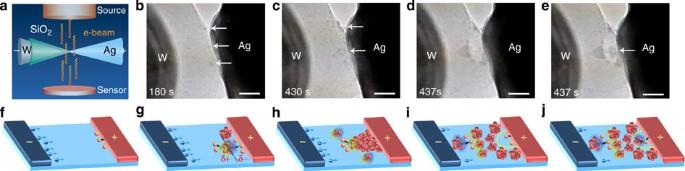Figure 4:In situTEM observation of bootstrapping filament growth and void formation. (a) Schematic of the experimental setup. (b–e) Real-time TEM images showing continuous filament growth within a 40-nm-thick SiO2film (applied voltage: 8 V). Scale bar, 20 nm. (f–j) Schematic illustration of the bootstrapping filament growth mode. (f) Ag ionization at the active electrode. (g) The nucleation of Ag nanoclusters near the active electrode. These nanoclusters act as bipolar electrodes in subsequent filament growth. (h) The growth of Ag nanoclusters at new positions that are closer to the inert electrode. (i) Migration of Ag nanoclusters leads to void formation marked by the dashed line. (j) Continued filament growth via step-by-step void refilling from the active electrode. Figure 4: In situ TEM observation of bootstrapping filament growth and void formation. ( a ) Schematic of the experimental setup. ( b – e ) Real-time TEM images showing continuous filament growth within a 40-nm-thick SiO 2 film (applied voltage: 8 V). Scale bar, 20 nm. ( f – j ) Schematic illustration of the bootstrapping filament growth mode. ( f ) Ag ionization at the active electrode. ( g ) The nucleation of Ag nanoclusters near the active electrode. These nanoclusters act as bipolar electrodes in subsequent filament growth. ( h ) The growth of Ag nanoclusters at new positions that are closer to the inert electrode. ( i ) Migration of Ag nanoclusters leads to void formation marked by the dashed line. ( j ) Continued filament growth via step-by-step void refilling from the active electrode. Full size image Additionally, a feature reminiscent of a void was observed in the SiO 2 film at the interface region in Fig. 4d,e , after large amounts of Ag atoms have passed through. The void formation is a clear sign of plastic deformation of the dielectric film due to increased mechanical stress that was introduced into the SiO 2 . Similar voids have also been observed for the cases of discrete nanoclusters (for example, Fig. 1j–l,p ). Apart from facilitating fast ion diffusion, the voids (channels) provide space for continuous movement of Ag clusters in a bootstrapping fashion as shown in Fig. 4d,e . As the existing Ag clusters move away towards the inert electrode new Ag clusters can move in and fill the void with reduced strain energy component (equation 1), facilitating the filament growth towards the inert electrode. The observation of the void channel formation and the dynamic step-by-step filament growth processes will be fundamentally important for the understanding and optimization of memristive device operations. Analysing the filament growth dynamics also reveals effects that can have significant practical implications for device operations. For example, Fig. 5a shows current–time ( I – t ) dependence of a Ag/SiO 2 /W device with a limited Ag source by reducing the contact area between the Ag electrode and the SiO 2 film. The corresponding dynamic filament growth TEM images are shown in Fig. 5b–f (also see Supplementary Movie 6 ). The device was initially in a high-resistance state and no filament growth was observed. At ~\n100 s, an abrupt resistive change was observed corresponding to the formation of conduction channel(s) inside the electrolyte (the dark region within the SiO 2 ) as shown in Fig. 5c,d . The filament formation, however, requires the consumption of the Ag electrode which serves as the Ag + ion supply. Notably, in Fig. 5a it was found that the current drops spontaneously after the initial filament formation. Close examination of the TEM recordings reveals that the current drop was due to the depletion of the Ag source (the Ag electrode) at the Ag/SiO 2 interface ( Fig. 5e,f ) leading to the breakage of the contact. This finding particularly is of critical significance for memristive device operations as the devices are scaled towards the 10 nm range. The depletion of electrode is less of a concern for large-scale devices with a virtually infinite Ag reservoir compared with the volume needed to form the filament (see Supplementary Fig. 1 , Supplementary Movie 7 , Supplementary Note 2 ). However, the consumption of the electrode material is no longer negligible when the device size is pushed close to the scaling limit, for example, where the electrode size is comparable with the filament size. For example, Supplementary Fig. 2 and Supplementary Movie 8 show that when the device size shrinks to 30–40 nm, the immediate contact to the filament at the Ag electrode/SiO 2 interface can be lost after the initial filament growth, even though overall electrical contact appears to be intact. 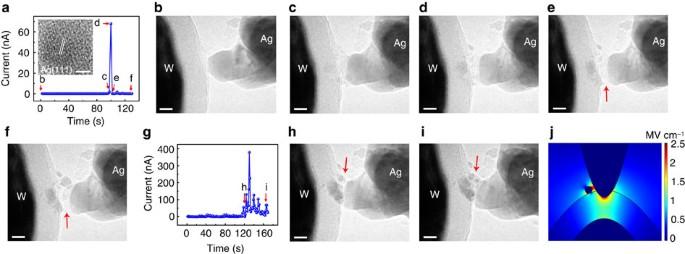Figure 5: Filament instability due to electrode depletion and recovery. (a)I–tcurve of the device. A constant voltage of 7 V was applied on the Ag electrode. The SiO2film thickness was 20 nm. The inset shows high-resolution transmission electron microscopy image of a Ag nanocluster inside the SiO2film, resolving (111) planes of Ag with a face-centered cubic (fcc) structure. Scale bar, 2 nm. (b–f) Real-time TEM images showing the filament growth at different stages corresponding to data points b–f ina. Scale bar, 10 nm. (g)I–tcharacteristics of the same device during reprogramming with a constant voltage of 2 V. (h,i) Real-time TEM images of the device corresponding to data points h, i ing, showing recovery of the Ag/SiO2contact. Scale bar, 10 nm. (j) Electric field distribution in the device state shown in (h,i) by COMSOL simulation. Figure 5: Filament instability due to electrode depletion and recovery. ( a ) I–t curve of the device. A constant voltage of 7 V was applied on the Ag electrode. The SiO 2 film thickness was 20 nm. The inset shows high-resolution transmission electron microscopy image of a Ag nanocluster inside the SiO 2 film, resolving (111) planes of Ag with a face-centered cubic (fcc) structure. Scale bar, 2 nm. ( b – f ) Real-time TEM images showing the filament growth at different stages corresponding to data points b–f in a . Scale bar, 10 nm. ( g ) I–t characteristics of the same device during reprogramming with a constant voltage of 2 V. ( h , i ) Real-time TEM images of the device corresponding to data points h, i in g , showing recovery of the Ag/SiO 2 contact. Scale bar, 10 nm. ( j ) Electric field distribution in the device state shown in ( h , i ) by COMSOL simulation. Full size image The broken electrical contact can be cured by refilling the gap at the Ag electrode/SiO 2 interface when positive voltage was continuously applied on the Ag electrode ( Fig. 5h,i , Supplementary Movie 9 ). The surface diffusion of atoms from the bulk of the Ag electrode into the gap was believed to drive this process, mediated by inhomogeneous electric field distribution around the gap [31] . Figure 5j shows the electric field distribution through a multiphysics simulation (Methods). A highly nonuniform electric field distribution is revealed and noticeably higher electric field intensity is seen in the vicinity of the nanogap, consistent with the observation that Ag atoms migrate towards the nano-gap region and refill the gap over time (see Supplementary Fig. 3 , Supplementary Note 3 ). Finally, we show that different growth modes can coexist in the same device when the growth dynamics can be properly tuned, as shown in Fig. 6 . After an initial growth period characterized by the step-by-step bootstrapping growth mode ( Fig. 6b–h , also see Supplementary Movie 10 ), the Ag clusters suddenly transformed into a much larger, dominant filament in Fig. 6i , accompanied by a significantly increase in current of >1 μA ( Fig. 6a ). Here the newly formed filament has a much wider base on the W cathode side and grows backwards towards the Ag electrode, and is much more solid, implying a transition to the conventional ECM growth mode shown in Fig. 3a . The structure of the new, solid filament was analysed using high-resolution transmission electron microscopy, where (111) planes of elemental Ag were clearly resolved ( Fig. 6j ) suggesting the filament corresponds to a crystalline Ag wire. The transition to the ECM mode (with high μ and Γ i ) can be explained by the increase of the device temperature due to the formation of the original filament, leading to significantly increased μ and Γ i (refs 18 , 32 ). The increase in Ag + ion mobility means that the ions have a much higher probability to reach the W cathode instead of piling inside the oxide through nucleation, as the increased temperature retards stable nucleus formation [33] . The combination of these effects suppresses the step-by-step cluster growth but enhances the rate of direct Ag + reduction at the W cathode, leading to the conventional ECM growth. 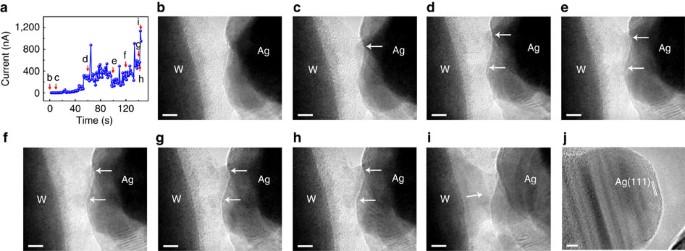Figure 6: Transition between different filament growth modes. (a)I–tcurve of the device with a 10-nm SiO2film. A constant voltage of 2 V was applied on the Ag electrode. (b–i) Real-time TEM images showing filament growth corresponding to data points b–i ina. Scale bar, 5 nm. (j) High-resolution transmission electron microscopy image of the filament iniafter removing the Ag electrode. Scale bar, 2 nm. The filament was found to be a solid crystalline Ag wire with face-centered cubic (fcc) structure. Figure 6: Transition between different filament growth modes. ( a ) I–t curve of the device with a 10-nm SiO 2 film. A constant voltage of 2 V was applied on the Ag electrode. ( b – i ) Real-time TEM images showing filament growth corresponding to data points b–i in a . Scale bar, 5 nm. ( j ) High-resolution transmission electron microscopy image of the filament in i after removing the Ag electrode. Scale bar, 2 nm. The filament was found to be a solid crystalline Ag wire with face-centered cubic (fcc) structure. Full size image To summarize, we report fundamental electrochemical dynamics of metal inclusions inside conventional solid-state dielectrics. The cluster interactions and formation processes are strongly affected by kinetic factors leading to different shapes and growth modes of the clusters that can be observed experimentally. Four types of metal systems and two types of device structures were studied, and based on these extensive experimental observations, we suggest a generalized framework governing the electrochemical dynamics of the metal clusters. The nanoclusters were found to act as BPEs under electric field, with their dissolution and nucleation processes mediated by the competing electrochemical reactions on both sides. By controlling the kinetic factors including ion mobility and redox rates, different growth modes can be achieved and verified experimentally. This framework well explains the apparently contradicting experimental observations of filament growth in memristive devices, and provides critical insight into the principle of device operations. Our qualitative model may help to develop a more quantitative and microscopic model for electric field-induced nanoionics based on two main kinetic factors, ion mobility and redox rate. These findings can be readily expanded to material and device systems where controlling the metal inclusion dynamics (or avoiding such) is critical and will have significant theoretical and practical impacts. in situ TEM The in situ TEM experiments were carried out using a Nanofactory scanning tunnelling microscopy platform inside a JEOL 3011 TEM operating at 300 kV. For samples with embedded metal clusters, the bottom electrode was grounded, while the top electrodes were individually addressed by the movable W probe, controlled by a piezomotor in the Nanofactory system. For the Ag/SiO 2 /W devices, the specimen was prepared by depositing a conformal SiO 2 film on a W probe (Bruker), and the probe was then mounted on the moveable end of a single-tilt TEM holder. A high-purity Ag wire (99.99%, Goodfellow) was fixed on the other end of the TEM holder, serving as the active electrode. The Ag/SiO 2 /W device structure was formed inside the TEM column when contact was achieved between the probe and the Ag wire. During in situ experiments on both types of devices, electrical signals were applied to the devices and measured through a low-noise Keithley 4200 semiconductor characterization system. The movies were recorded simultaneously with the electrical measurements. Preparation of FIB samples The TEM specimens with embedded Ag, Cu, Ni and Pt metal nanoclusters were prepared by FIB. First, Au films (400 nm) with a NiCr adhesion layer (20 nm) were deposited on SiO 2 /Si substrates by electron beam evaporation, serving as the bottom electrodes. Afterwards, a SiO 2 layer with a thickness of ~\n20 nm was evaporated, followed by the evaporation of thin Ag, Cu, Ni or Pt metal layers. A second SiO 2 layer with a similar thickness of ~\n20 nm was then evaporated. The samples were then subjected to rapid thermal annealing processes in Ar. The metal layers form nanoclusters embedded in the SiO 2 films during annealing when the metal film is thin enough (~\n1 nm). Afterwards, a 100-nm thick Au film was evaporated to form the top electrode. The TEM specimens were then prepared out of these samples by successive FIB lift-out, patterning and thinning processes. The devices were designed in such a configuration that all the devices in the same sample have individual top electrodes while sharing the bottom electrode. The lift-out, patterning and thinning processes were conducted on a dual-beam FIB system (FEI Helios Nanolab 650 FIB workstation). During FIB patterning, low-energy Ga + milling with extreme care was used to obtain high-quality and thin TEM specimens in order to reduce the projection effect caused by cluster distributions in the Z direction. Preparation of samples on W probes Silicon dioxide films were deposited on W tips in high vacuum at a low evaporation rate of 0.01 nm s −1 by electron beam evaporation. The SiO 2 film thickness was adjusted in the range of 10–50 nm. The samples were checked by TEM, and the SiO 2 films were found to be fully conformal. Simulations Electric field simulations were performed using a COMSOL multiphysics package based on finite element analysis. Simulations on cluster movement dynamics via splitting and merging processes were performed using a custom Matlab code based on equations (2, 3) by assuming for the nanocluster downstream. The two interacting nanoclusters were modelled by perfect spheres with a constant total volume, and the maximum distance between the two spherical surfaces (from the leftmost position on the left sphere to the rightmost position on the right sphere) was assumed fixed when their diameters vary during the electrochemical oxidation and reduction processes. How to cite this article: Yang, Y. et al. Electrochemical dynamics of nanoscale metallic inclusions in dielectrics. Nat. Commun. 5:4232 doi: 10.1038/ncomms5232 (2014).